Azoarene activation for Schmidt-type reaction and mechanistic insights The Schmidt rearrangement, a reaction that enables C-C or C-H σ bond cleavage and nitrogen insertion across an aldehyde or ketone substrate, is one of the most important and widely used synthetic tools for the installation of amides and nitriles. However, such a reaction frequently requires volatile, potentially explosive, and highly toxic azide reagents as the nitrogen donor, thus limiting its application to some extent. Here, we show a Schmidt-type reaction where aryldiazonium salts act as the nitrogen precursor and in-situ- generated cyclopenta-1,4-dien-1-yl acetates serve as pronucleophiles from gold-catalyzed Nazarov cyclization of 1,3-enyne acetates. Noteworthy is that cycloketone-derived 1,3-enyne acetates enabled ring-expansion relay to access a series of 2-pyridone-containing fused heterocycles, in which nonsymmetric cycloketone-derived counterparts demonstrated high regioselectivity. Aside from investigating the scope of this Schmidt-type reaction, mechanistic details of this transformation are provided by performing systematic theoretical calculations. Nitrogen-based heterocycles constitute the basic structural scaffold of substantial bioactive natural products and are present in approximately half of marketed drugs, with nonplanar heterocycles featuring five- and/or six-membered ring frameworks being of great interest to the fields of pharmaceutical discovery, chemical biology, and medical chemistry [1] , [2] , [3] , [4] , [5] . Especially abundant among these heterocycles are those incorporating a 2-pyridinone framework, a privileged structure that is composed of the core of many alkaloids exhibiting potent biological activities (Fig. 1a ) [6] , [7] , [8] , [9] , [10] , [11] . Consequently, the development of innovative strategies for the assembly of 2-pyridone-containing heterocycles has been a hot research topic in the organic community [12] , [13] , [14] . The Schmidt reaction represents a long-standing popular nitrogenation approach to furnish these aza-heterocycles from cyclic ketones with HN 3 or alkyl azides [15] , [16] , [17] , [18] , [19] . However, its dependence on volatile, highly toxic, and potentially explosive azide reagents offers great possibilities for further exploration [20] , [21] , [22] (Fig. 1b ). Despite the astonishingly persistent efforts on hydrazoic acid replacements, the use of azide still prevails in this field [23] , [24] , [25] . The Beckmann rearrangement starting from cyclic oximes has been recognized as a well-known alternative pathway to approach cyclic amides [26] , [27] . However, typically catalytic Beckmann rearrangements often require some specialized active cyclic oximes, strong Brønsted acids, or preactivation of the hydroxyl (e.g., by tosylation) [28] , [29] , [30] , [31] , thus limiting the potential application to some extent. Ideally, if one easily available and widespread chemical could be activated by a suitable catalytic system while endowed with new reactivity [32] , [33] , [34] , [35] , [36] , [37] , it would advance innovative chemical technology that influences broad fields of academia and industry. Fig. 1: Azoarene activation for the Schmidt reaction. a Natural products and bioactive molecules containing 2-pyridinone structures. b Traditional Schmidt reaction with azides as the limiting reagent. c Reactivity patterns of aryldiazonium salts. d Our study on 2-pyridinone synthesis via the sequence involving Nazarov cyclization, nucleophilic addition, and Schmidt reaction. Full size image Because of their highly electrophilic character and moderate oxidizability, aryldiazonium salts, easily prepared from the corresponding anilines, demonstrate broad-spectrum reactivities and are often used as both aryl precursors and dinitrogen proelectrophiles in numerous transformations, such as the Meerwein arylation [38] , [39] , cross-coupling reactions [40] , [41] , [42] , [3 + 2] annulation [43] , [44] , and Japp-Klingemann reaction [45] , [46] , [47] . In the well-known Japp-Klingemann procedure, the addition of cyclic ketones into aryldiazonium salts produces rather unstable azo compounds, which are converted into hydrazones via 1,3-hydrogen transfer (Fig. 1c ) [45] , [46] , [47] . In contrast, the reactivity of aryldiazonium salts as a nitrogen donor for the Schmidt reaction remains unknown. We hypothesized that the key to realizing the Schmidt reaction is to suppress the 1,3-hydrogen transfer process in the Japp-Klingemann procedure. Therefore, the removal of the proton at the α-position of azoarenes for migration while exploiting the intrinsic nucleophilicity of azoarenes may provide a feasible scheme for the Schmidt reaction. Homogeneous gold catalysis has been acknowledged as an effective strategy for constructing functional molecules in synthetic chemistry benefited from the impressive characteristics of its high catalytic capabilities, high levels of regioselectivity, and mild reaction conditions as well as good functional group tolerance [48] , [49] , [50] , [51] , [52] , [53] . The gold-catalyzed Nazarov cyclization of nucleophilic 1,n-enyne acetates toward cyclopenta-1,4-dien-1-yl acetates is among the more exploited reactions [54] , [55] , [56] , [57] , [58] , [59] , [60] , [61] . However, to date, there are only a few reports that deal with the inherent nucleophilicity of in-situ generated cyclopenta-1,4-dien-1-yl acetates toward intermolecular nucleophilic substitution reactions [55] , [58] . In sharp contrast, the nucleophilic addition of this intermediate remains elusive. Along this line, we believe that highly electrophilic aryldiazonium salts could be trapped by in-situ-generated nucleophilic cyclopenta-1,4-dien-1-yl acetates to access the azo intermediate, which facilitates acyl transfer and the subsequent rearrangement process for the Schmidt-type reaction (Fig. 1d ). Thus, this cascade activation strategy would demonstrate simple and available aryldiazonium salts as a cyclic nitrogenated partner akin to azides, but with remarkable elimination of associated hazards. In this work, we report that gold-catalyzed transformation of 1,3-enyne acetates with aryldiazonium salts enables merging Nazarov cyclization with a Schmidt-type reaction for the general synthesis of valuable 2-pyridinone-based heterocyclic systems as well as synthetically appealing azasteroid chemistry (Fig. 1d ). Of note is that the gold complex could be compatible with aryldiazonium salts without observation of their redox transformation with each other. Intrigued by the ring-expansion relay and high regioselectivity observed in nonsymmetric cycloketone-derived 1,3-enyne acetates, we carefully performed systematic theoretical calculations to elucidate the catalytic cycle for σ-bond migration, the azoarene activation mode and the influence on the regioselectivity (see the mechanism section and Supplementary Information ). Reaction optimization To test our initial hypothesis, we began by studying the gold-catalyzed reaction of 1,3-enyne acetates and aryldiazonium salts as test substrates to develop straightforward access to highly functionalized cyclopenta[ c ]pyridin-1-ones, which are classically synthesized via catalytic cyclization reactions that exhibit a lack of flexibility [62] , [63] , [64] . 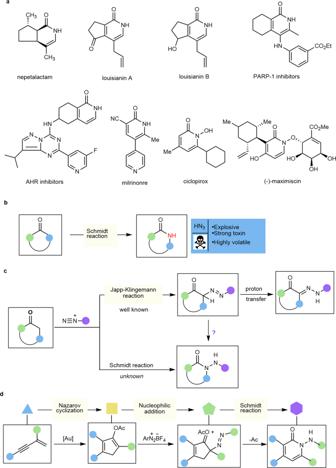Fig. 1: Azoarene activation for the Schmidt reaction. aNatural products and bioactive molecules containing 2-pyridinone structures.bTraditional Schmidt reaction with azides as the limiting reagent.cReactivity patterns of aryldiazonium salts.dOur study on 2-pyridinone synthesis via the sequence involving Nazarov cyclization, nucleophilic addition, and Schmidt reaction. Diverse gold catalysts and solvents were evaluated at room temperature for 6 h, as shown in Table 1 . To our delight, by using JohnPhosAu(MeCN)SbF 6 (1.0 mol %) as a catalyst, the reaction of strained cyclobutanone-derived 1,3-enyne acetate 1a with 2a in 1,2-dichloroethane (DCE) afforded cyclopenta[ c ]pyridin-1-one product 3 in 65% yield through a Schmidt-type reaction (entry 1). Several other gold catalysts widely used in catalytic transformations, such as Ph 3 PAuCl, XPhosAuCl, SPhosAuCl, IPrAuNTf 2 , AuCl 3 , and AuCl, were then examined (entries 2–7). The results revealed that all these catalysts could drive the transformation to the desired product 3 except for SPhosAuCl, and the former two led to moderate yields of product 3 (entries 2–3); in contrast, the latter three demonstrated very poor catalytic capabilities and provided lower yields (<29%, entries 5–7). Taking JohnPhosAu(MeCN)SbF 6 as the catalyst, we then investigated the effect of the solvent by exploiting toluene, tetrahydrofuran (THF), acetone, and DCM (entries 8–11). However, the use of the former two was almost ineffective, as only a trace amount of product 3 was detected (entries 8–9). The reaction independently proceeded in the latter two solvents, but both gave unsatisfactory results associated with the reaction yields in comparison to DCE (entries 10–11 vs entry 1). This reaction could run at higher temperatures, but gave a slightly complex system and a decrease in yields was detected (entries 12–13). Table 1 Optimization conditions for forming 3 a Full size table Evaluation of the substrate scope With these acceptable reaction conditions (Table 1 , entry 1), we set out to systematically investigate the scope of this transformation by examining the behaviors of 1,3-enyne acetates and aryldiazonium salts. The results are summarized in Fig. 2 . First, aryldiazonium salts associated with various substituents successfully participated in this gold-catalyzed ring-expansion relay with 1a , orienting regiospecific access to the desired cyclopenta[ c ]pyridin-1-ones 4–18 in good yields (Fig. 2 ). Both electron-donating (EDG) (e.g., methyl, 2b − 2d ) and electron-withdrawing (EWG) (e.g., fluoro, 2e ; chloro, 2f − 2h ; bromo, 2i ; trifluoromethyl, 2j ; cyano, 2k , and nitro, 2l ) groups at different positions ( ortho , meta , or para ) demonstrated good compatibility of this transformation. Of these functional groups, both o -tolyl ( 2b ) and o -chlorophenyl ( 2f ) analogs with strong steric congestion were well-tolerated with this catalytic system, illustrating that the increased steric hindrance had little influence on the reactivity. In addition, three strong electron-withdrawing groups such as CF 3 , CN, and NO 2 at the para -position remained highly reactive in this catalysis, delivering the targets 12–14 in 67–75% yields. Furthermore, the protocol was also compatible with naphthalen-2-yl counterpart 2m . Notably, three derivatives of naturally occurring chiral alcohol-based esters (L(-)-borneol ( 2n ), L-menthol ( 2o ), and 1-adamantanol ( 2p )) were also applicable, producing corresponding products 16–18 in good yields through two carbon-carbon bond cleavages. In addition to the cyclobutanone-derived substrate, less strained cyclopentanone-derived counterpart 1b worked readily, enabling a similar catalytic ring-expansion/nitrogen insertion process to deliver functionalized tetrahydroisoquinolin-1(2H)-ones 19–34 in synthetically useful yields (Fig. 2 ). Next, the potential variations in the structure of 1,3-enyne acetates were further examined, with p -chlorophenyl substrate 2h as the other partner. 1,3-Enyne acetate 1c , which bears a phenyl group at the C3 position of the cyclobutene ring, afforded desired product 35 in good yield. 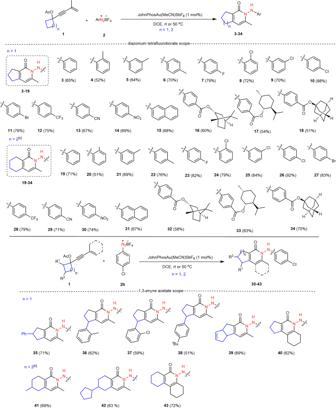Fig. 2: Schmidt-type reaction for the synthesis of bicyclic 2-pyridinones. Reaction conditions:1(0.2 mmol),2(0.4 mmol), JohnPhosAu(MeCN)SbF6(1 mol%), DCE (2.0 ml), room temperature (rt), 6 h; the yield refers to isolated yield based on1; use of cyclopentyl acetate1is at 50 °C. Importantly, this ring-expansion reaction proceeded with complete regioselectivity when aryl substituents were installed into the C2 position of the cyclobutene ring, in which a less steric methylene group is more prone to migrate than methine functionality with a substituent under gold-catalyzed conditions. As exemplified by 1,3-enyne substrates 1d–1f , the expected products 36–38 as single regioisomers were isolated, albeit with moderate yields. A similar phenomenon was discovered in the transformations of both bicyclo[3.2.0]hept-2-en-6-one-derived ( 1g ) and C2-alkylated cyclopentanone-derived ( 1i and 1j ) substrates, and regioisomeric products 39 , 41 and 42 were generated with good yields. Moreover, internal alkynes 1h and 1k that bear a cyclohexenyl substituent were still tolerated, providing tricyclic products 40 and 43 in acceptable yields (Fig. 2 ). Fig. 2: Schmidt-type reaction for the synthesis of bicyclic 2-pyridinones. Reaction conditions: 1 (0.2 mmol), 2 (0.4 mmol), JohnPhosAu(MeCN)SbF 6 (1 mol%), DCE (2.0 ml), room temperature (rt), 6 h; the yield refers to isolated yield based on 1 ; use of cyclopentyl acetate 1 is at 50 °C. Full size image After the success of the catalytic ring-expansion relay reactions of formal cycloketone-derived 1,3-enyne acetates and aryldiazonium salts, we proceeded to examine other types of naturally occurring cycloketone derivatives, and therefore offer a general ring-expansion strategy to build up other N -heterocycles incorporating two medicinally relevant privileged core structures. Azasteroids, normally derived from chemical modifications of steroids, are recognized as a privileged pharmacophore prevalent in pharmaceutical agents [65] , [66] , but relatively few approaches to their syntheses have been documented in recent years [67] , [68] , [69] . We questioned whether steroid-derived 1,3-enyne acetates could be included in our catalytic cycle as pro-nucleophilic partners to react with aryldiazonium salts 2 . If successful, this reaction would demonstrate an efficient and regiospecific approach to form pentacyclic azasteroid motifs. Following this idea, we tested the reaction of estrone-derived 1,3-enyne acetate 1l with aryldiazonium salt 2d under the optimized conditions (Table 1 , entry 1). To our delight, the desired pentacyclic azasteroid 44 was obtained in 59% yield (Fig. 3 ). Furthermore, an array of electron-withdrawing groups, such as halo, trifluoromethyl, cyano, and nitro substituents, at the para -position of the benzene ring of aryldiazonium salts proved to be compatible with this protocol (Fig. 3 ). In addition, epiandrosterone-derived substrate 1m (tetrahydropyran protection) could be utilized to react with aryldiazonium salts, furnishing diversely substituted azasteroids 50–51 in good yields (Fig. 3 ). Fig. 3: Schmidt-type reaction for the synthesis of azasteroids. Reaction conditions: 1 l or 1 m (0.2 mmol), 2 (0.4 mmol), JohnPhosAu(MeCN)SbF 6 (1 mol%), DCE (2.0 ml), 50 °C, 6 h; the yield refers to isolated yield based on 1 . Full size image To further expand the utility of this methodology, we devoted our effort to testing aldehyde-derived 1,3-enynes as pro-nucleophiles for pyridin-2(1 H )-one synthesis, because such compounds are a class of prevalent heteroaromatic structures that are frequently encountered in a broad variety of natural products, bioactive agents and approved drugs [70] , [71] , [72] . For this reason, reactions of aldehyde-derived 1,3-enyne acetates with aryldiazonium salts were carried out under standard conditions, and used to produce a wide range of pyridin-2(1 H )-ones 52-70 with generally good yields in a regiospecific manner (Fig. 4 ). Aromatic aldehyde-derived 1,3-enyne acetates 1n-1w bearing both electron-donating and electron-withdrawing groups, regardless of their positions, could be readily engaged in the reaction. Various functional groups, including methyl ( 1o–1q ), halogens (Cl, 1r–1t and F, 1 u ), and trifluoromethyl ( 1v ), were compatible with this catalytic system. The naphthalene ring ( 1w ) was also exclusively installed into the product ( 61 ). As exemplified by substrate 1x , this protocol was also adaptable to the 1,3-enyne acetate attached to a heteroarene such as thiophene in an acceptable yield ( 62 , 51%). Moreover, switching the aryl group at the α-position of 1,3-enyne substrates to other substituents, such as cycloalkyl (cyclopropyl 1 y and cyclohexyl 1z ), benzyl ( 1aa ), branched ( 1ab ) and linear ( 1ac ) alkyl, and cinnamyl ( 1ad ), had a negligible effect on the reaction performance, orienting the complete regioselectivity to access the target pyridin-2(1 H )-one products 63-68 with acceptable yields. When the methyl group (R 3 ) on the terminal alkene moiety of 1,3-enyne acetates was replaced by phenyl and n -pentyl groups, products 69 and 70 were isolated in 68% and 73% yields, respectively. Then, we examined the generality of this catalytic annulation/nitrogen insertion cascade regarding aryldiazonium salts 2 by combining with benzaldehyde-derived substrate 1n . The detailed investigations on substituents including alkyl, halogens, trifluoromethyl, cyano, and nitro at different positions in the arene ring as well as a sterically more demanding bicyclic aromatic example, such as naphthyl group, revealed that all these attempts were applicable for the reaction (products 71–82 , Fig. 4 ). The presence of halogen, cyano, and nitro moieties in these synthons adds greatly to the synthetic value of the cyclization products, as they can act as an additional handle for late-stage transformations. Aryldiazonium salts that bear a chiral alcohol-based ester such as L(-)-borneol ( 2n ), L-menthol ( 2o ), 1-adamantanol ( 2p ) and (-)-isopulegol ( 2q ) on the benzene ring successfully gave corresponding products 83–86 in 56-65% yields (Fig. 4 ). Fig. 4: Schmidt-type reaction for the synthesis of poly-substituted 2-pyridinones. Reaction conditions: 1 (0.2 mmol), 2 (0.4 mmol), JohnPhosAu(MeCN)SbF 6 (1 mol%), DCE (2.0 ml), room temperature (rt), 6 h; the yield refers to isolated yield based on 1 . Full size image Gram-scale synthesis and synthetic applications To demonstrate the practicality and scalability of the present protocol, gram-scale reactions of 1a and 1o (5.0 mmol) and 2k were independently carried out with 1 mol% JohnPhosAu(MeCN)SbF 6 under the optimized conditions, affording products 11 and 78 in slightly diminished yields (Fig. 5 a, b ). Subsequently, compound 11 reacted with methyl iodide in the presence of NaH, furnishing methyl-protected 87 in 78% yield (Fig. 5a ). Treatment of 78 with Br 2 gave polybrominated product 88 in 82% yield, followed by the Ir-catalyzed reaction of tetramethyldisilazane (TMDS) to access 3,5-dibromopyridin-2(1H)-one 89 in 62% yield through N-N bond cleavage (Fig. 5b ). A similar transformation occurred when using 78 and TMDS in the presence of iridium catalyst (Fig. 5b ). Fig. 5: Gram-scale experiments and synthetic applications. a Gram-scale synthesis of 11 and N -protection of 11 . b Gram-scale synthesis of 78 and synthetic transformations. TMDS, tetramethyldisilazane. Full size image Mechanistic studies To gain mechanistic insights into this nitrogen insertion process, some control experiments were conducted, as shown in Fig. 6 . In Zhang’s procedure, gold-catalyzed Nazarov cyclization of 1,3-enyne acetates led to two different products of cyclopentenones and unstable cyclopentadienes [54] . To investigate the possibility of intermediates for this reaction, a gold-catalyzed reaction of 1a was run under standard conditions for 1 h, and then 2a was placed into this reaction system. As a result, instead of the target 3 , 2-methyl-3,4,5,6-tetrahydropentalen-1(2 H )-one 91 was generated, along with the recovered 2a (Fig. 6a ). Without a gold catalyst, the reaction between preformed 2-methyl-3,4,5,6-tetrahydropentalen-1-yl acetate 92 and 2a gave a 50% yield of 3a (Fig. 6b ). Next, treatment of 92 with 2a under standard conditions provided a slightly increased yield (56%, Fig. 6c ). These outcomes demonstrate that cyclopentadienes, rather than cyclopentenones, are potential reaction intermediate, and the gold catalyst is unnecessary but could promote the nitrogen insertion reaction to some extent. Let us examine in detail the roles of tetrafluoroborate anion and H 2 O (Fig. 6d ). Without tetrafluoroborate, the reaction of 1a with benzenediazonium chloride did not proceed under the standard conditions whereas the use of 2.0 equivalents of silver tetrafluoroborate as tetrafluoroborate sources provided 3a in 58% yield. Exchanging silver tetrafluoroborate for silver acetate did not give 3a . The reaction in the absence of H 2 O also did not work. Evidently, when 1.0 equivalent of H 2 O was added to the above reaction system, product 3a was obtained in 61% yield. These results indicate that both tetrafluoroborate and H 2 O are crucial for this transformation (for their roles, see the mechanism section). Fig. 6: Preliminary mechanism investigations. a Two-step reaction of 1a with 2a . b Metal-free reaction of 92 with 2a . c The role of the gold catalyst in the Schmidt-type reaction. d Investigations on the roles of tetrafluoroborate anion and H 2 O for Schmidt-type reaction. Full size image Possible reaction pathways To investigate the possible mechanism of the Au(I)-catalyzed Schmidt-type reaction between cyclopentadienyl acetate and aryldiazonium salt, a theoretical study employing density functional theory (DFT) calculations was performed at M06-L/def2-TZVPP/SMD dichloroethane //M06-L/def2-SVP/SMD dichloroethane level of theory [73] (Fig. 7 ). As a typical π-acetic metal, Au in active species catalyst could be coordinated by cyclopentadienyl acetate 1g to form complex M1 with exergonic energy of 8.4 kcal/mol. Activated by the π-acetic Au(I) cation, the coordinating C-C triple bond could be nucleophilically attacked by the intramolecular ester group to achieve stepwise acetoxy transfer via the six-membered ring transition states TS1 and TS2 . The corresponding free energy barriers are 12.1 kcal/mol and 2.8 kcal/mol, respectively, indicating a rapid process. The consequence of stepwise acetoxy transfer is the formation of oxonium intermediate M3 , which could be regarded as an equilibrium with intermediate M1 in thermodynamic [74] , [75] , [76] . 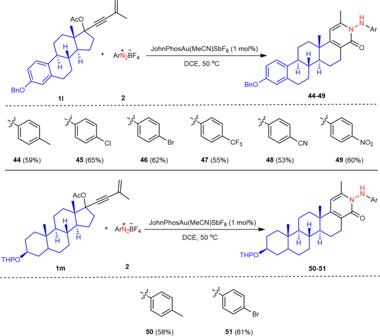Fig. 3: Schmidt-type reaction for the synthesis of azasteroids. Reaction conditions:1lor1m(0.2 mmol),2(0.4 mmol), JohnPhosAu(MeCN)SbF6(1 mol%), DCE (2.0 ml), 50 °C, 6 h; the yield refers to isolated yield based on1. Resonance structure M3’ clearly reveals the electrophilicity of its terminal methylene position, which results in an intramolecular electrophilic 1,5-annulation via transition state TS3 to irreversibly form an Au-carbene complex M4 . The calculated free energy barrier for the step was detected to be 13.7 kcal/mol. The resonance structure of M4’ reveals a cationic carbon, which would cause 1,2-carbon cation rearrangement. The calculated free energy barrier for the intramolecular 1,2-shift of the unsubstituted methyl group via transition state TS4 is 10.1 kcal/mol. However, the corresponding energy barrier of the cyclopentyl shift via transition state TS5 is 17.8 kcal/mol. Therefore, fused pentalenyl acetate M5 was found to be the major product, which is fully consistent with the experimental observations. Fig. 7: Calculated free energy profiles for the cationic Au(I) catalyzed cyclization of cyclopentadienyl acetate. 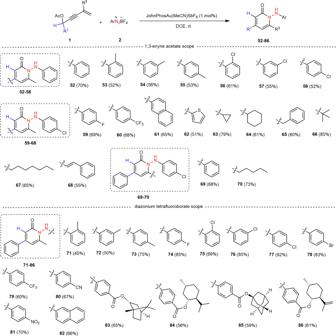Fig. 4: Schmidt-type reaction for the synthesis of poly-substituted 2-pyridinones. Reaction conditions:1(0.2 mmol),2(0.4 mmol), JohnPhosAu(MeCN)SbF6(1 mol%), DCE (2.0 ml), room temperature (rt), 6 h; the yield refers to isolated yield based on1. The relative free energies are computed at the M06-L/def2-TZVPP/SMD dichloroethane //M06-L/def2-SVP/SMD dichloroethane level. Full size image To further analyze the regioselectivity, the Newman projections of transition states TS4 and TS5 are given in Fig. 8 . In the geometry of transition state TS4 , the strain of the fused five-membered ring (right part) promoted the rotation of the projecting C-C single bond, which led to the 1,2-shift of the methyl group with strain release. Meanwhile, the corresponding projecting C-C bond in TS5 is free without strain. Therefore, the lack of a driving force makes the corresponding 1,2-shift difficult via TS5 . Fig. 8: The Newman projected structure of the transition states TS4 and TS5. The torsion angles are computed at the M06-L/def2-TZVPP/SMD dichloroethane //M06-L/def2-SVP/SMD dichloroethane level. Full size image The reaction pathway of further transformation of fused pentalenyl acetate M5 was also considered by DFT calculations. As shown in Fig. 9 , the enol ester moiety of M5 could nucleophilically attack aryldiazoniom salt 2 h via transition state TS6 affording oxonium intermediate M7 with a free energy barrier of only 18.6 kcal/mol. After that, two possible pathways for the expansion of the ring could occur: acyl transfer promoted arrangement (solid black lines) or nitrogen-insertive expansion (dashed red lines). In intermediate M7 , the azo moiety reveals nucleophilicity, which can attack the acyl group to achieve an intramolecular acyl transfer via transition state TS7 with a free energy barrier of only 9.7 kcal/mol. The acyldiazenium moiety in intermediate M8 leads to the cleavage of an active C-C bond via transition state TS8 with an energy barrier of only 0.8 kcal/mol. The generated carbonyl cation in intermediate M9 could undergo an intramolecular nucleophilic attack by carbonyl cation via transition state TS9 , which provides an oxodihydropyridinium intermediate M10 . Furthermore, a deprotonation process could be associated with a complex of water and BF 4 anion via transition state TS10 with a free energy barrier of only 6.7 kcal/mol. Finally, the stepwise hydrolysis of Ac-protected product M11 could lead to the formation of the final product P-39 . Moreover, resonance structure M7’ exhibits an electrophilic carbon atom, which can be nucleophilically attacked by an azo moiety via transition state TS13 to afford aziridinium intermediate M13 . Although C-C bond cleavage via transition state TS14 , hydrolysis of amide and deprotonation could also provide the same product P-39 , the much higher free energy barrier of this process makes it an unfavorable path. Fig. 9: Calculated free energy profiles for the cyclization of aryldiazonium salt and intermediate 3 H -cyclopenta[ a ]pentalen-1-yl acetate M5. The relative free energies are computed at the M06-L/def2-TZVPP/SMD dichloroethane //M06-L/def2-SVP/SMD dichloroethane level. Full size image In this work, the discovery of a Schmidt-type reaction triggered by the soft nucleophilicity of azoarenes is described. This provides a general and practical approach to highly substituted 2-pyridinones and their fused heterocyclic system from readily available 1,3-enyne acetates with aryldiazonium salts in a highly regioselective fashion. The reaction is catalyzed by a well-defined air-stable gold catalyst, involving a 3,3-rearrangement/Nazarov cyclization and nitrogen insertion pathway, under mild conditions and demonstrates wide substrate compatibility. Mechanistic studies reveal a soft nucleophilic property of azoarenes to induce C-C cleavage and nitrogen insertion. Systematic theoretical calculations led us to propose that ring strain controls the regioselectivity of C-C σ-bond migration for nonsymmetric cycloketone-derived 1,3-enyne acetates and that the nucleophilicity of azoarenes induces acyl migration to achieve Schmidt-type rearrangement, thereby giving rise to 2-pyridinone-based cyclic products with high annulation efficiency and regioselectivity from unsaturated linear substrates. 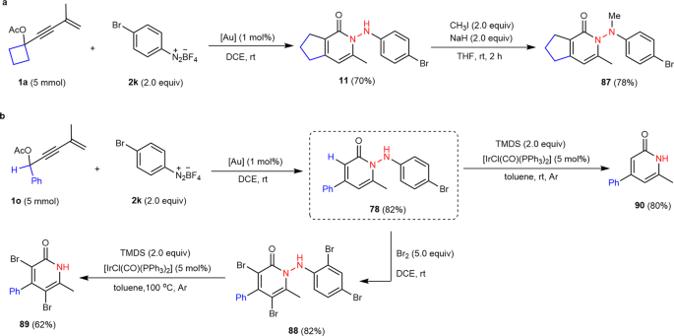Fig. 5: Gram-scale experiments and synthetic applications. aGram-scale synthesis of11andN-protection of11.bGram-scale synthesis of78and synthetic transformations. TMDS, tetramethyldisilazane. General procedure for the gold-catalyzed domino reaction of 1,3-enyne acetates and aryldiazonium tetrafluoroborates. To a 10 mL Schlenk tube under air conditions, cyclobutanone- and aldehyde-derived 1,3-enyne acetates ( 1 , 0.2 mmol), aryldiazonium tetrafluoroborates ( 2 , 0.4 mmol), JohnPhosAu(MeCN)SbF 6 (1 mol%), and 1,2-dichloroethane (2.0 ml) were successively added. 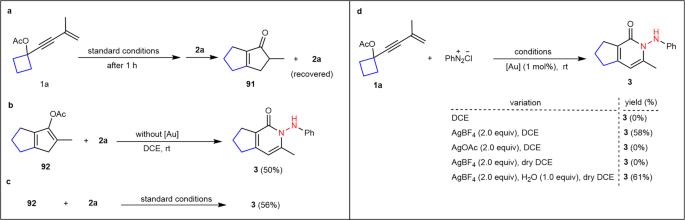Fig. 6: Preliminary mechanism investigations. aTwo-step reaction of1awith2a.bMetal-free reaction of92with2a.cThe role of the gold catalyst in the Schmidt-type reaction.dInvestigations on the roles of tetrafluoroborate anion and H2O for Schmidt-type reaction. 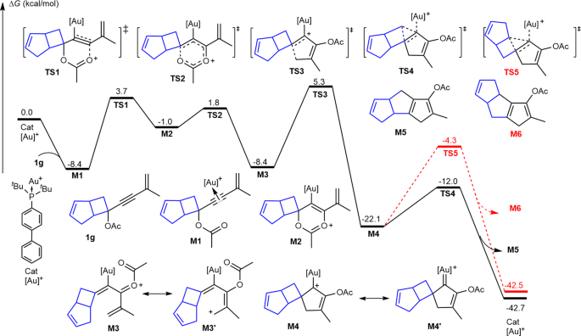Fig. 7: Calculated free energy profiles for the cationic Au(I) catalyzed cyclization of cyclopentadienyl acetate. The relative free energies are computed at the M06-L/def2-TZVPP/SMDdichloroethane//M06-L/def2-SVP/SMDdichloroethanelevel. 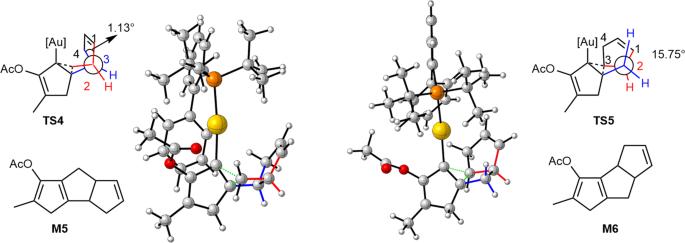Fig. 8: The Newman projected structure of the transition states TS4 and TS5. The torsion angles are computed at the M06-L/def2-TZVPP/SMDdichloroethane//M06-L/def2-SVP/SMDdichloroethanelevel. 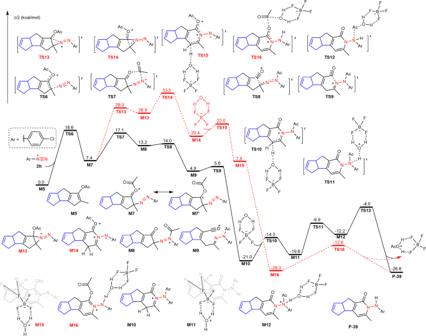Fig. 9: Calculated free energy profiles for the cyclization of aryldiazonium salt and intermediate 3H-cyclopenta[a]pentalen-1-yl acetate M5. The relative free energies are computed at the M06-L/def2-TZVPP/SMDdichloroethane//M06-L/def2-SVP/SMDdichloroethanelevel. The mixture was stirred at room temperature (the reaction of cyclopentanone-derived 1,3-enyne acetates was at 50 °C) for 6 h. After the reaction was completed (indicated by TLC, petroleum ether: ethyl acetate = 2:1), the reaction mixture was concentrated by vacuum distillation and was purified by flash column chromatography to afford the desired pure products 3–86 .